The missing boundary in the phase diagram of PbZr1−xTixO3 PbZr 1−x Ti x O 3 (PZT) is one of the most important and widely used piezoelectric materials. The study of its local and average structures is of fundamental importance in understanding the origin of its high-performance piezoelectricity. Pair distribution function analysis and Rietveld refinement have been carried out to study both the short- and long-range order in the Zr-rich rhombohedral region of the PZT phase diagram. The nature of the monoclinic phase across the Zr-rich and morphotropic phase boundary area of PZT is clarified. Evidence is found that long-range average rhombohedral and both long- and short-range monoclinic regions coexist at all compositions. In addition, a boundary between a monoclinic (M A ) structure and another monoclinic (M B ) structure has been found. The general advantage of a particular monoclinic distortion (M A ) for high piezoactivity is discussed from a spatial structural model of susceptibility to stress and electric field, which is applicable across the wide field of perovskite materials science. Piezoelectric materials are used in a large variety of applications including actuators, sensors, electromechanical motors and sonar systems. The global market for piezoelectric actuators and motors was projected to reach $12.3 billion in 2014 with an annual growth rate of 13.2% per year, according to a report [1] published in 2010. One of the most widely used piezoelectric ceramic materials (around 98% of the total actuator market) is the solid solution of lead zirconate (PbZrO 3 ) and lead titanate (PbTiO 3 ), commonly known as PZT, with general formula PbZr 1− x Ti x O 3 . This material belongs to the class of crystal structures known as perovskites with formula ABX 3 , where A and B are cations and X is an anion, usually oxygen. The fundamental structure (known as the aristotype) is cubic in space group , with the anions forming a corner-linked array of octahedra. The A cation occupies the space between the octahedra while the B cation is at the centre of the octahedra. The importance of this structure is that it can occur in many subtle structural modifications that have significant effects on the properties of the material. Such structures are highly pseudosymmetric. For instance the cations can be displaced off-centre by relatively small amounts in various directions and if cations (of type A and/or B) are all displaced in the same general direction the crystal may show polar properties such as piezoelectricity, pyroelectricity or ferroelectricity. In addition, the anion octahedra can tilt [2] about various directions to create many different ‘puckered’ structures, sometimes combined with cation displacements. This wealth of structural variations with corresponding physical properties leads to perovskites having many industrial applications, and to understand the origin of their physical properties it is important to investigate their crystal structures. There is also considerable interest in finding new piezoelectrics that do not contain toxic elements such as lead. However, to date there are still no lead-free piezoelectrics in production on a widespread industrial scale that have better performance and versatility than the Pb-based materials. To overcome this situation, we first need to understand the origin of high piezoelectricity in PZT, which is still not clear largely because of PZT’s structural complexity. Studies of the average (long-range) structure over nearly 60 years have revealed new phenomena while at the same time leaving problems that remain unsolved. As part of this, recent attention has been paid to the short-range scale structural complexity of PZT and its relationship to the piezoactivity. Total scattering and pair distribution function (PDF) methods have developed rapidly during the past decades, helping to reveal the complex local structure of many functional materials [3] . In this paper, we combine PDF analysis and conventional average structure analysis methods to explore the short-range and long-range structures of PZT. It should be explained that here the term ‘short-range’ refers to a situation where the correlation length between any pair of atoms in a structural array of atoms is sufficiently short (possibly a few nanometres) that the determination of the crystal structure using the sharp Bragg peaks in an X-ray, neutron or electron diffraction pattern would result in an average structure with some atoms occupying disordered positions. The term ‘long-range’ refers to a correlation length that is long enough that the sharp Bragg scattering would lead to determination of a crystal structure that is fully ordered. PZT displays a complicated temperature-composition phase diagram [4] , including the so-called morphotropic phase boundary (MPB) at x ≈0.48. The piezoelectric properties appear as Ti is added to PbZrO 3 from about x =0.08 and increase continuously until reaching a maximum at x ≈0.45–0.48 (refs 5 , 6 , 7 ). The MPB was originally believed to be a near vertical line in the phase diagram separating the Ti-rich tetragonal (T) region (in space group P 4 mm ) and Zr-rich rhombohedral (R) regions. The R region consists of two ferroelectric rhombohedral phases, existing at low and high temperature. At low temperature the space group is R 3 c and the crystal structure is characterized by cation displacements along the pseudocubic [111] direction, together with oxygen octahedral tilting of the type a - a - a - (ref. 2 ). At higher temperature the space group becomes R 3 m, retaining the cation displacements but losing the octahedral tilts. The symmetries of the R and T phases are not group–subgroup related, and for many years it was not understood how such an MPB could exist. An intermediate monoclinic (M) phase (space group Cm ), which is a subgroup of R 3 c, R 3 m and P 4 mm, was discovered by Noheda et al. [8] and this finding has now been generally accepted. One explanation for the high piezoelectric response based on this model was then given by a first-principles calculation by Bellaiche et al. [9] and experimentally studied by Guo et al. [10] This is known as the polarization-rotation model, in which the displacements of the Pb atom are free to change orientation within a mirror plane in each unit cell, as allowed by the M-phase symmetry. This mechanism was also found in other Pb-based piezoelectrics, such as Pb(Zn 1/3 Nb 2/3 )O 3 -PbTiO 3 (ref. 11 ). An alternative macroscopic model that stresses the role of domains [12] , [13] , has also been proposed, for which some experimental evidence [14] exists. In all likelihood both models have a part in the piezoelectric response. However, while the phase boundary between M and T phases has always been distinct, the boundary between the R and M regions has never been experimentally observed, and this has raised questions over the existence of the R phase itself. Furthermore, a number of diffraction experiments on PZT structures have shown that over a large compositional range outside the MPB region PZT ceramics consist of a mixture of M and other phases [15] , [16] , [17] , [18] , [19] . In the neutron and X-ray diffraction refinements of the R phase by several researchers [20] , [21] , [22] , the least-squares refined anisotropic displacement parameters indicated that the Pb atom density distribution was disk-shaped with the disk perpendicular to [111]. This was explained by displacing the Pb atoms away from the rhombohedral threefold axes to create local monoclinic structures [22] that averaged to an overall rhombohedral symmetry. On the basis of this assumption, Glazer et al. [23] further proposed that the different average structures of PZT (R, M and T) could all be described in terms of local monoclinic ordering. Near the MPB region, the formation and the growth of these nanoscale regions may then account for the enhanced piezoactivity, in support of a domain-controlled contribution to the high piezoelectric properties [24] , [25] . An alternative suggestion to explain the missing boundary between R and M phase regions was made by Pandey et al. [26] , who proposed that there is no rhombohedral phase at all and that the apparent disordering of the Pb atoms arose from refining the structure in too high a symmetry. This model implied that the whole R region was really long-range monoclinic in space group Cm or Cc . While such a picture might be attractive, our own studies using neutron diffraction and Rietveld refinement failed to support this idea, instead indicating that there is a mixture of R and M phases present for most compositions, including within the MPB region [15] , [16] , [27] . It should be borne in mind that Rietveld refinement of mixed pseudosymmetric phases, including those of low symmetry, pushes the Rietveld analysis to its limits, because of the increased number of refinable parameters. Nonetheless, we believe that our mixed-phase refinements are valid. First of all this is because the refined compositions follow a distinct and understandable trend [16] with composition. Furthermore, in the original refinement of Corker et al. [22] , which did not consider the possibility of mixed phases and, moreover, used diffraction data of lower resolution than in the later mixed-phase refinements, it was observed that the Pb displacement decreased on approaching the MPB. Such behaviour is surprising given that the piezoelectric effect increases towards the MPB. In the mixed-phase refinements, however, we found that the Pb displacements did not decrease. Differences between short- and long-range ordering for the oxygen atoms have also been observed above the Curie temperature [28] , [29] . However, although there has been some published work regarding the real local structures of PZT [30] , [31] , [32] , [33] , [34] , [35] , most lack a thorough analysis of the role of the Pb atoms in the MPB area. Here, PDF analyses of PZT compositions with x =0.2, 0.3 and 0.4 are presented and a re-examination of earlier Rietveld results show that the displacements of the Pb atoms undergo a composition-enforced change between two monoclinic variants, thus revealing a monoclinic–monoclinic boundary (crossover) for the first time. Definition of PDF Total neutron scattering data were collected at room temperature to study the local structure of PZT in the Zr-rich compositions away from the MPB ( x =0.2, 0.3, 0.4) where we know that the Pb and O disorder is most significant. On average, it is well accepted that within the R region, the Pb and Zr/Ti cations are displaced, on average, along the threefold [111] axis, with respect to pseudocubic axes. There is to date no evidence of any ordering of the Zr and Ti atoms. In the work of Corker et al. [22] , Zr and Ti atom displacements were refined separately with the Zr displacement values found to be much smaller than those for Ti. However, the ability of Rietveld refinement to make such fine distinctions in two separate overlapping atomic positions is unreliable, and so in most refinements, these two atoms have been treated to be displaced equally in the average structure. The Pb atom displacement lengths are about three times those of Zr/Ti for all the compositions [16] . The PDF is the sine Fourier Transform of the total scattering data, and expresses the probability of finding two individual atoms separated by a distance r in real space [36] . With the help of the well-developed Reverse Monte Carlo (RMC) method [37] , [38] , one can extract information about the local structure from the PDF data. For the three individual compositions, we used a starting model of 10 × 10 × 10 pseudocubic unit cells with 5,000 atoms, on the basis of the Rietveld-refined average structure, and then performed a large number of RMC iterations against the experimental PDF, total scattering S (Q) and Bragg profile data. Periodic boundary conditions were used throughout. We estimated the effect of different model sizes to determine the error in total radial distribution function G (r). For 5 × 5 × 5 the error was 8.1%, while for 10 × 10 × 10 it was 1.3% and for 15 × 15 × 15 it was 1.3%. Comparison between PDFFIT and RMC The PDF data for the three compositions were first compared with the PDF patterns refined from the average structures of R and M symmetries using the software PDFFIT [39] . 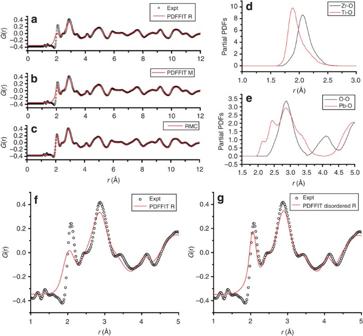Figure 1: Comparison with experimental results. (a) PDFFIT forx=0.3 at room temperature using a rhombohedral structure, (b) using a monoclinic structure. (c) Fitting by Reverse Monte Carlo method. (d) Low-rpartial PDF peaks for Zr-O and Ti-O. (e) Low-rpartial PDF peaks for Pb-O and O-O from the RMC modelling. (f) Enlargement ofFig. 1ashowing the disagreement between the observed and fitted results. (g) Addition of disordered Pb displacements around the [111] axis now gives rise to the shoulders on the main Pb-O peak (PDF/RMC plots forx=0.2, 0.3 and 0.4 are available in theSupplementary Figs 1–5). Figure 1a,b show the comparison for x =0.3 as an example, where significant differences, especially at low r , are apparent. The positive Zr-O and negative Ti-O peaks can be seen (the neutron scattering length for Ti is negative) at 2.08 Å and 1.80 Å, respectively. This difference in Zr-O and Ti-O bond lengths is consistent with the difference between Zr and Ti ionic radii (15–30 pm). Figure 1c shows that RMC modelling gives an excellent fit to the observed data. Partial PDFs for these two types of bond further show different peak shapes ( Fig. 1d ). The peak shape for the Zr-O bonds is symmetric and corresponds with these bonds being closely equal in length, which cannot be explained by any polar structure. A similar phenomenon was also observed in the PDF analysis by Dmowski et al. [31] and in EXAFS studies by Cao et al. [33] On the other hand, the Ti-O peak is asymmetric showing Ti is displaced along the [111] direction. This shows that, in addition to the Pb displacements, the Ti displacements contribute more to the electric polarization than the Zr displacements, confirming that Ti is a more ferroelectrically active B-site cation than Zr. Figure 1: Comparison with experimental results. ( a ) PDFFIT for x =0.3 at room temperature using a rhombohedral structure, ( b ) using a monoclinic structure. ( c ) Fitting by Reverse Monte Carlo method. ( d ) Low- r partial PDF peaks for Zr-O and Ti-O. ( e ) Low- r partial PDF peaks for Pb-O and O-O from the RMC modelling. ( f ) Enlargement of Fig. 1a showing the disagreement between the observed and fitted results. ( g ) Addition of disordered Pb displacements around the [111] axis now gives rise to the shoulders on the main Pb-O peak (PDF/RMC plots for x =0.2, 0.3 and 0.4 are available in the Supplementary Figs 1–5 ). Full size image In Fig. 1a,b , another key feature to note is in the region from 2.3 Å to 3.7 Å. The experimental data show a strong peak at 2.88 Å with shoulders on each side, which are not seen in the PDFFIT simulation for both R and M symmetries. The sums of the Pb-O and O-O bonds form a complex pattern in this region, and the shoulders are mainly due to the Pb-O partial PDF ( Fig. 1e ), showing that either the average long-range R 3 c / R 3 m or Cm / Cc structures alone cannot completely explain the short-range Pb-O correlation. The shoulders on the Pb-O peak in Fig. 1e are explained by placing the Pb atoms in a disordered arrangement around the [111] direction at distances varying from 0.05 to 0.3 Å, but lying on the three symmetry-related mirror planes. Figure 1g confirms that the shoulders are accounted for by this model, provided that the displacements are not all the same size: at this composition the Rietveld refinements [15] show that there is a significant fraction of monoclinic phase mixed with the rhombohedral phase, and so this explains why the threefold symmetry for the Pb displacements has to be broken. Evidence for two phases To analyse the element-specific local structural details, the displacements of the cations (Pb, Zr, Ti) were calculated using the method of Keeble et al. [40] measured from the average centres of the surrounding oxygen polyhedral cages based on the RMC models obtained. The distributions of the atomic displacement directions were then plotted in the form of stereographic projections. 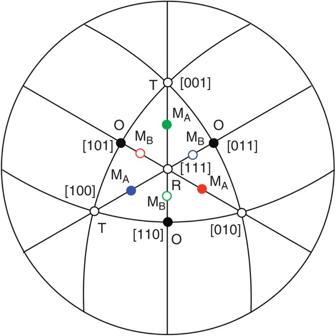Figure 2: Stereographic projection for a pseudocubic perovskite viewed down [111]. The average cation displacement directions: along the [111] axis for rhombohedral (R), on the {110} mirror planes for monoclinic phases MA(red, green and blue full circles) and MB(red, green and blue hollow circles) and along the <001> axes for tetragonal (T) are marked individually. The black dots marked O on the <110> directions refer to orthorhombic symmetry. For clarity, only the central region of the stereographic projection is marked. Figure 2 shows a pseudocubic stereographic projection down [111] with the possible directions for the cation displacement vectors marked for R, orthorhombic (O), T and M phases. If the structure is rhombohedral, the cations are displaced along the [111] axis, marked R on the figure. There are two possible monoclinic phases of interest here denoted M A and M B according to the notation of Vanderbilt and Cohen [41] , where the atomic displacements lie within {110} mirror planes. The difference between these two monoclinic phases is simply that the M A phase has cation displacements between the R and T positions, whereas the M B phase is between R and O positions. Figure 2: Stereographic projection for a pseudocubic perovskite viewed down [111]. The average cation displacement directions: along the [111] axis for rhombohedral (R), on the {110} mirror planes for monoclinic phases M A (red, green and blue full circles) and M B (red, green and blue hollow circles) and along the <001> axes for tetragonal (T) are marked individually. The black dots marked O on the <110> directions refer to orthorhombic symmetry. For clarity, only the central region of the stereographic projection is marked. Full size image The displacement directions of the Zr and Ti as modelled using RMC are very different. Stereographic projections representing the Zr and Ti displacement directions ( Fig. 3 ) confirm that Zr displacement directions are highly disordered while the Ti displacement directions cluster tightly around the [111] rhombohedral symmetry axis for all compositions studied. This is also supported by the slightly larger peak width for the Zr-O partial PDF peak ( Fig. 1d ); the FWHMs for the Ti-O and Zr-O peaks are 0.15 Å and 0.20 Å, respectively. When the Ti concentration increases to x =0.4 ( Fig. 3 ), Zr becomes almost completely disordered with only a small quantity of atomic displacements clustered around the [111] axis. 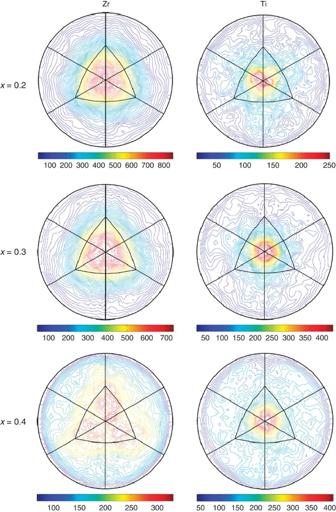Figure 3: Stereographic projections for B-cation displacements. Depicted are the cases forx=0.2, 0.3 and 0.4 viewed down [111]. Figure 3: Stereographic projections for B-cation displacements. Depicted are the cases for x =0.2, 0.3 and 0.4 viewed down [111]. Full size image The statistical distribution of the Pb displacement directions for PZT is plotted on a stereographic projection in Fig. 4 for angles close to the [111] direction. Most of the Pb displacements are not distributed around a distinctly separate point on the monoclinic mirror plane, which means that in this composition range there is no evidence for a single long-range monoclinic structure as proposed by Pandey et al. [26] Instead, the structural data point to the PZT material being a mixture of an average rhombohedral structure with disordered Pb displacements plus a long-range monoclinic structure. This is consistent with our Rietveld [15] refinement results where we found that in addition to a rhombohedral phase there was also a long-range monoclinic Cm component. 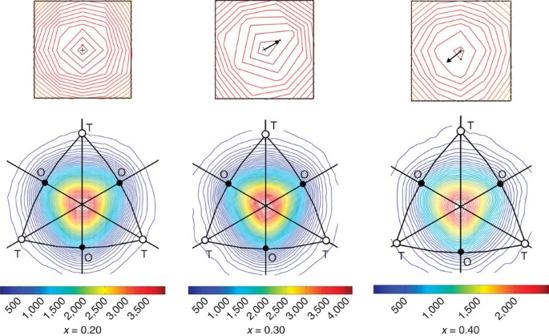Figure 4: Stereographic projections of Pb atom displacements. The projections forx=0.2, 0.3 and 0.4, show the presence of local monoclinic phases with different Pb distributions on the monoclinic mirror planes at MAand MBpositions in addition to displacements along the rhombohedral axis. The insets are magnifications of the central areas with arrows indicating displacement directions away from [111] marked by a cross. (SeeFig. 2for definition of directions). To decrease the error, displacements <0.3 Å have been eliminated. Figure 4: Stereographic projections of Pb atom displacements. The projections for x =0.2, 0.3 and 0.4, show the presence of local monoclinic phases with different Pb distributions on the monoclinic mirror planes at M A and M B positions in addition to displacements along the rhombohedral axis. The insets are magnifications of the central areas with arrows indicating displacement directions away from [111] marked by a cross. (See Fig. 2 for definition of directions). To decrease the error, displacements <0.3 Å have been eliminated. Full size image Evidence for two monoclinic phases For x =0.2, the distribution is relatively isotropic, and this is consistent with the fact that at this composition the Rietveld results [15] , [22] indicate that most of the ceramic is rhombohedral with disordered Pb atomic positions. However for x =0.3, a small shift of the centre of gravity of the distribution is found along a mirror plane to a position lying between the R and O points. Such a displacement is consistent with the existence of a monoclinic component of the type M B . For x =0.4, on the other hand, the Pb distribution is displaced along the R–T direction, consistent with the presence of a fraction of M A phase. This suggests the following model for the structures in this region. Much of the material consists of an average rhombohedral structure with short-range local monoclinic Pb displacements. In addition the correlation length of these monoclinic regions spans a range from the unit cell level (as in the rhombohedral fraction) up to much larger correlations to the extent that they create a coexisting long-range monoclinic phase of symmetry Cm . 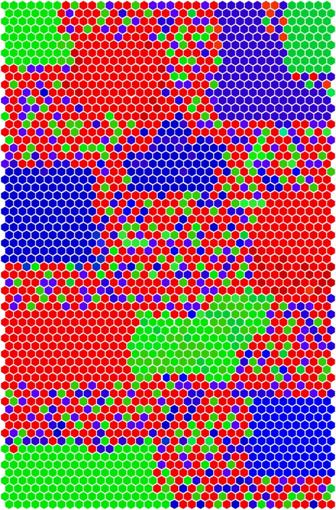Figure 5: Schematic view of short and long-range ordered regions of monoclinic symmetry unit cells. Viewed down the [111] pseudocubic direction, the three colours, red, green and blue refer to three possible Pb orientations as in the stereographic projection inFig. 2. No distinction is made here between MAand MBstructures. A detailed description can be found in the text. Figure 5 is a schematic diagram viewed down the [111] direction, illustrating the structural arrangement envisaged. Three colours (red, green and blue) are used to indicate the three possible monoclinic unit cells (Pb atoms on three mirror planes in space group Cm as either M A or M B ). Part of the structure consists of large ordered regions, which would give rise to distinct monoclinic diffraction patterns (for Bragg scattering to be observed these regions would in fact have to be considerably larger than can be shown in this diagram, although smaller regions would also be expected). Also in the figure are regions with short-range correlations of monoclinic unit cells, which give rise to a diffraction pattern of average rhombohedral symmetry. Of course, this division between rhombohedral and monoclinic structures could be between different grains or as implied in Fig. 5 , within a single crystal grain. Figure 5: Schematic view of short and long-range ordered regions of monoclinic symmetry unit cells. Viewed down the [111] pseudocubic direction, the three colours, red, green and blue refer to three possible Pb orientations as in the stereographic projection in Fig. 2 . No distinction is made here between M A and M B structures. A detailed description can be found in the text. Full size image Our observation that at x =0.4 there is some M A phase present is entirely consistent with the discovery by Noheda et al. [8] However what was entirely unexpected is the observation that for x =0.3 there is evidence for the presence of some M B phase. Note that both M A and M B phases have the same Cm space group and are distinguished only by the direction of the Pb displacements. The separate observation of M A and M B phases in different compositions of PZT led us to re-examine our earlier Rietveld refinements, where for x <0.48, there is a coexistence of rhombohedral and monoclinic phases [15] , [16] (Full details of the structural parameters for each composition are to be found in Supplementary Table 1 ). For the monoclinic fraction at each composition, we first determined the centroid of the 12 oxygens coordinating the Pb atom and then found the Pb displacement from this point. This enabled us to calculate the angles between the [111] direction and the Pb displacement directions on the monoclinic mirror plane in the Cm phase, defined as negative when rotating towards M B directions, that is, [110], positive when rotating towards M A directions, that is [001]. In agreement with the indications from the RMC model, the results show that at room temperature the Pb atoms are displaced in the M B directions for x ~<0.35. The Pb displacement direction then rotates within the mirror plane, through [111], between x =0.30 and 0.35, corresponding to the M A phase on further increasing Ti concentration ( Fig. 6 ). At the PbZrO 3 end of the phase diagram ( x <0.08) there is an antiferroelectric orthorhombic space group Pbam [42] phase (O). Now finally viewing the whole PZT phase diagram through the lens provided by the Pb displacement directions ( Fig. 6 ), we see a progression from the O phase to the M B phase, which crosses to the M A phase through [111], and then through the MPB to the T phase. This plot suggests that the actual crossover between the two monoclinic structures may be discontinuous. 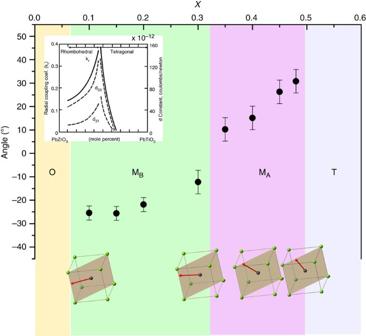Figure 6: Pb displacement angles. The angles are calculated away from the [111] direction as a function of Ti concentration at room temperature on the basis of Rietveld refinement15,16(the full set of Rietveld data is given inSupplementary Table 1). The bottom figures illustrate the Pb displacement directions in the monoclinic phases that coexist with the rhombohedral phase. Note that the range of angles permissible lie between −35.3° (towards the orthorhombic phase) and 54.7° (towards the tetragonal phase). The inset shows the piezoelectric measurements of Jaffeet al.(Reprinted with permission from ref.5. Copyright 1954, AIP Publishing LLC). Figure 6: Pb displacement angles. The angles are calculated away from the [111] direction as a function of Ti concentration at room temperature on the basis of Rietveld refinement [15] , [16] (the full set of Rietveld data is given in Supplementary Table 1 ). The bottom figures illustrate the Pb displacement directions in the monoclinic phases that coexist with the rhombohedral phase. Note that the range of angles permissible lie between −35.3° (towards the orthorhombic phase) and 54.7° (towards the tetragonal phase). The inset shows the piezoelectric measurements of Jaffe et al. (Reprinted with permission from ref. 5 . Copyright 1954, AIP Publishing LLC). Full size image The missing boundary The Pb displacement angles at different temperatures and for different compositions ( Fig. 7 ) indicate a slightly curved boundary corresponding to the crossover between M A and M B structures. The observed monoclinic ( Cm symmetry) structure can be thought of as an extension of the short-range components of the rhombohedral fraction to the longer range. Our study of the Pb displacement direction in the monoclinic fraction has revealed a hitherto unobserved boundary. The Rietveld refinement results [15] have shown that the monoclinic phase fraction increases on approaching the MPB [16] from the Zr-rich end. We can now explain that this monoclinic fraction is initially composed of the M B phase, which exists on a variety of length scales. The short-range component looks rhombohedral on average, whereas the long-range component is observed as the monoclinic phase. As x increases, the correlation lengths of the short-range M B components grow so that correspondingly more monoclinic phase is seen (and less rhombohedral phase). As x approaches 0.30 to 0.35, the long-range M B phase converts to M A , the fraction of which continues to increase and become dominant at the MPB. As such this means that there is no distinct R–M boundary to be found. Our observation of a regular change in the Pb displacement directions is consistent with the recent discovery that the different phases are mainly controlled by a single mode [43] . It also adds further support that the original mixed-phase Rietveld refinements are meaningful, despite the large number of refinable parameters. 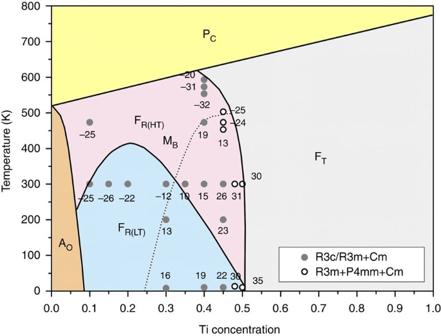Figure 7: The new phase diagram for PZT. The diagram superimposes the angles between the directions of the Pb displacements and the [111] direction. The crossover between MBand MAstructures is marked by a dashed line. The marked phase regions are cubic PC, orthorhombic AOand the ferroelectric phases tetragonal FT, rhombohedral FR(LT)and rhombohedral FR(HT),using the notation of Jaffeet al.4 Figure 7: The new phase diagram for PZT. The diagram superimposes the angles between the directions of the Pb displacements and the [111] direction. The crossover between M B and M A structures is marked by a dashed line. The marked phase regions are cubic P C , orthorhombic A O and the ferroelectric phases tetragonal F T , rhombohedral F R(LT) and rhombohedral F R(HT), using the notation of Jaffe et al. [4] Full size image This M A −M B crossover has never been observed before in ceramic PZT or in related compounds. It is very subtle and it is a moot point as to whether one should call this a true phase boundary or not. Our study shows why it has been so difficult to observe until now as these two monoclinic structures both belong to the same space group and give powder diffraction patterns that are virtually the same. Furthermore, the ceramics in these composition ranges consist of mixtures of long-range rhombohedral and monoclinic phases, thus complicating structural refinement. It also shows that the true width of the MPB region at room temperature, as defined by the presence of the M A phase, extends from about x =0.35 to 0.48, considerably broader than in earlier suggestions. The curve of Pb displacement directions in Fig. 6 becomes steeper with composition in the M A region thus indicating that the Pb displacement would be more sensitive to change by external fields or stress than in the M B region; hence, a rapid increase in piezoelectric response should be expected, as is indeed observed (inset to Fig. 6 ). It is easy to see why this is so by reference to the space available for the Pb atoms to change displacement direction in the crystal structure. For the M A arrangement ( Fig. 8 ), the Pb atom can rotate its displacement direction between [001] and [111] whereas in M B it can rotate from [111] to [110] (see Supplementary Movie 1 , an animated GIF showing this rotation). The latter encompasses a smaller angle than that available for the former and so the M A phase enables the Pb displacement more ‘room’ to be affected by an external stress or field. Furthermore the increase in the amount of long-range monoclinic phase with Ti content also would increase the response of the ceramic to external fields. It is clear that to obtain maximum piezoresponse in a perovskite solid–solution system such as PZT, it is preferable to have the M A structure rather than M B . This distinction between the importance of M A and M B phases has not been stressed hitherto and is an outcome of general importance in the wide field of perovskite materials science. 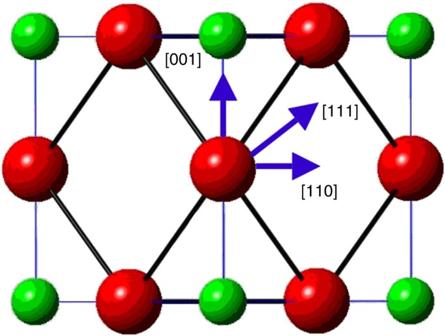Figure 8: Pb displacements in the perovskite structure. Viewed along thedirection, the illustration shows the available space for the displacement directions to be changed. Figure 8: Pb displacements in the perovskite structure. Viewed along the direction, the illustration shows the available space for the displacement directions to be changed. Full size image Sample preparation and neutron PDF measurement Ceramic samples were prepared by the conventional mixed oxide method. The details of sample preparation conditions can be found in Yokota et al. [15] The total neutron scattering experiments were carried out at ISIS (Rutherford Appleton Laboratory) on GEM (General Materials Diffractometer). High-quality data were obtained up to a Q of 50 Å −1 , and were corrected for attenuation, inelasticity effects, multiple scattering and background using the standard Gudrun software. RMC modelling was implemented using the package RMCProfile [44] , [45] . The total radial distribution function G (r), the corrected total scattering structure factors S (Q) and the Bragg profile data were fitted together with bond valence sum constraints and realistic distance window constraints. To improve the statistics of the results, the data for each composition were modelled 60 times. Stereographic projections Construction of the stereographic projections was made in the following way. First of all unit cells within the total array where the number of oxygens coordinating the cations was incorrect were omitted from the calculation. The displacement directions were then computed for remaining unit cells, in 5° angular steps with averaging over a range of 8°. In this way, a smooth plot is achieved. Neutron powder diffraction The neutron powder diffraction measurements were performed at ISIS on HRPD (High-Resolution Powder Diffractometer) at various temperatures. Rietveld refinement was carried out using TOPAS Academic [46] . The data were collected using the high-angle back-scattering bank detectors, which provide the d-spacing range ~0.3–2.2 Å. The scale factor, background parameters, peak-shape function parameters, absorption and strain parameters were refined in all cases. How to cite this article: Zhang, N. et al. The missing boundary in the phase diagram of PbZr 1−x Ti x O 3 . Nat. Commun. 5:5231 doi: 10.1038/ncomms6231 (2014).